Dispersed cells represent a distinct stage in the transition from bacterial biofilm to planktonic lifestyles Bacteria assume distinct lifestyles during the planktonic and biofilm modes of growth. Increased levels of the intracellular messenger c-di-GMP determine the transition from planktonic to biofilm growth, while a reduction causes biofilm dispersal. It is generally assumed that cells dispersed from biofilms immediately go into the planktonic growth phase. Here we use single-nucleotide resolution transcriptomic analysis to show that the physiology of dispersed cells from Pseudomonas aeruginosa biofilms is highly different from those of planktonic and biofilm cells. In dispersed cells, the expression of the small regulatory RNAs RsmY and RsmZ is downregulated, whereas secretion genes are induced. Dispersed cells are highly virulent against macrophages and Caenorhabditis elegans compared with planktonic cells. In addition, they are highly sensitive towards iron stress, and the combination of a biofilm-dispersing agent, an iron chelator and tobramycin efficiently reduces the survival of the dispersed cells. Bacteria are able to switch between the planktonic and biofilm modes of growth. In contrast to the free living, planktonic mode, biofilm bacteria aggregate and embed themselves in a self-generated matrix consisting of extracellular polymeric substances, with the entire complex often (but not necessarily) attached to a surface [1] . Acute infections are, in general, caused by planktonic cells, which can be successfully treated via the administration of antibiotics. Chronic infections are believed to involve bacteria in biofilms. The host immune system and conventional antimicrobials often fail to eradicate such infections [2] , [3] , [4] . It is estimated that biofilms are responsible for 65–80% of the infections occurring in the human body [5] , which, due to their persistence and chronic nature, place a massive burden on healthcare systems worldwide. Through dispersal processes, biofilms can spark new infections within the host and result in the transmission of bacteria between different hosts [4] , [6] . One medically relevant biofilm-forming bacterium is the opportunistic pathogen Pseudomonas aeruginosa , which is primarily known for its involvement in cystic fibrosis [7] , catheter-related infections [8] , and eye [9] and chronic wound infections [10] . Bis-(3′-5′)-cyclic dimeric GMP (c-di-GMP) is an essential secondary messenger that many bacterial species employ in the control of biofilm formation and dispersal [11] . The intracellular content of c-di-GMP is determined by diguanylate cyclases that catalyse the formation of c-di-GMP and phosphodiesterases (PDEs) that degrade c-di-GMP [11] . Bacterial cells can adjust their intracellular c-di-GMP content rapidly to adapt to complex and changing environmental conditions. During exposure to stress, including starvation and nitrosative conditions, bacterial cells can reduce their intracellular c-di-GMP content by activating specific PDEs, resulting in biofilm dispersal [12] , [13] , [14] . The active process of dispersing cells is specific and regulated, in contrast to mechanical and passive dispersal, which involves sloughing off biofilm cells. While it is common knowledge that biofilm cells differ from dispersed cells [15] , it is unclear whether biofilm-dispersed cells are similar to planktonic cells with respect to their physiology. In addition to biofilm dispersal, there is increasing evidence that PDEs are involved in the pathogenicity of bacteria [16] , [17] , [18] . In line with this evidence, we have recently demonstrated that a low intracellular c-di-GMP content increases the resistance of P. aeruginosa to antimicrobial peptides [19] . Macrophages have been shown to rapidly reduce the intracellular content of c-di-GMP of engulfed uropathogenic Escherichia coli [20] . This finding suggests a link between dispersed cells with low c-di-GMP and increased virulence. Here, we seek to elucidate whether there is a unique physiology associated with freshly dispersed biofilm cells. We use single-nucleotide resolution transcriptomic analysis to compare the gene expression profiles of biofilm-dispersed cells with those of planktonic and biofilm cells of P. aeruginosa . We show that the type II secretion system (T2SS) is induced in the biofilm-dispersed cells and that the dispersed cells can kill macrophages and escape phagocytosis. In addition, dispersed cells are more lethal to Caenorhabditis elegans compared with planktonic bacteria. Furthermore, there is a huge reduction in the expression of genes involved in iron stress responses in biofilm-dispersed cells compared with planktonic and biofilm cells. Combining an iron chelator and biofilm-dispersing agents results in the improved eradication of biofilm-dispersed cells. The present study has implications for future intervention strategies based on chemically mediated biofilm dispersal. Dispersed cells represent a distinct stage of bacterial life We were able to generate dispersed cells from biofilms of P. aeruginosa through the reduction of intracellular c-di-GMP either chemically, by applying sodium nitroprusside (SNP), or enzymatically, by inducing the expression of a plasmid-encoded YhjH PDE [19] . SNP is a nitric oxide-releasing compound that induces biofilm dispersal via the activation of the PDE DipA [21] . The chemical and enzymatic dispersals of P. aeruginosa biofilms showed similar dispersal dynamics ( Fig. 1a ). Dispersed cells from P. aeruginosa biofilms possessed lower levels of c-di-GMP ( Fig. 1b ) and the major siderophore pyoverdine compared with planktonic cells ( Fig. 1c,d ). To investigate the stability of the dispersed cells, we monitored their pyoverdine levels continuously in ABTGC medium, in 0.9% NaCl, and in ABTGC medium containing dispersal agents. We found that the dispersed cells maintained their low-pyoverdine phenotype in 0.9% NaCl or in ABTGC medium dispersal agents ( Fig. 1c,d ). In growth medium without dispersal agents, the dispersed cells first exhibited a 2-h lag phase. Then, they initiated growth, and their pyoverdine levels rapidly increased to the level observed in planktonic bacteria ( Fig. 1c,d ). These experiments suggested that dispersed cells reverted to planktonic cells after 2 h and that the dispersed cell phenotype was maintained in the presence of dispersing agents. The population of the dispersed cells was highly homogenous. After a 5-h induction of dispersal, more than 95% of the dispersed cells still exhibited low expression levels of the pyoverdine synthesis gene pvdA , according to the confocal image analysis of bacteria carrying a pvdA - gfp reporter ( Fig. 1e ). This result suggested that there were only a few planktonic cells mixed with the dispersed cells. In the experiments described below, the dispersed cells were maintained in a medium with dispersal agent to maintain their phenotype. 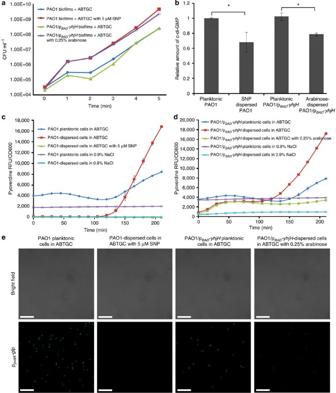Figure 1: Generation of biofilm-dispersed cells. (a) Biofilm dispersal dynamics monitored by colony-forming units. Biofilms of PAO1 and PAO1/pBAD-yhjHwere dispersed in ABTGC medium supplied with 5 μM SNP and 0.25% arabinose, respectively. Control experiments were performed using ABTGC medium without SNP or arabinose. Means and s.d. from triplicate experiments are shown. (b) Relative intracellular c-di-GMP of planktonic cells and dispersed cells determined by high-performance liquid chromatography. Means and s.d. from triplicate experiments are shown. *P<0.05, Student’st-test. (c) Reversion of SNP-dispersed cells in ABTGC, 0.9% NaCl and ABTGC supplied with 5 μM SNP. SNP-dispersed cells were inoculated into microplates containing ABTGC, 0.9% NaCl or ABTGC supplied with 5 μM SNP, respectively, and monitored for their pyoverdine fluorescence by using a Tecan Infinite Pro2000 microplate reader. Means and s.d. in relative fluorescence units (RFU) from triplicate experiments are shown. (d) Reversion ofyhjH-dispersed cells in ABTGC, 0.9% NaCl and ABTGC supplied with 0.25% arabinose.YhjH-dispersed cells were inoculated into microplates containing ABTGC, 0.9% NaCl or ABTGC supplied with 0.25% arabinose, respectively, and monitored for their pyoverdine fluorescence using a Tecan Infinite Pro2000 microplate reader. Means and s.d. in RFU from triplicate experiments are shown. (e) Expression of the ppvdA-gfpfusion in planktonic cells and dispersed cells after 5-h dispersal. Representative confocal images are shown for each condition. Scale bars, 10 μm. Figure 1: Generation of biofilm-dispersed cells. ( a ) Biofilm dispersal dynamics monitored by colony-forming units. Biofilms of PAO1 and PAO1/p BAD -yhjH were dispersed in ABTGC medium supplied with 5 μM SNP and 0.25% arabinose, respectively. Control experiments were performed using ABTGC medium without SNP or arabinose. Means and s.d. from triplicate experiments are shown. ( b ) Relative intracellular c-di-GMP of planktonic cells and dispersed cells determined by high-performance liquid chromatography. Means and s.d. from triplicate experiments are shown. * P <0.05, Student’s t -test. ( c ) Reversion of SNP-dispersed cells in ABTGC, 0.9% NaCl and ABTGC supplied with 5 μM SNP. SNP-dispersed cells were inoculated into microplates containing ABTGC, 0.9% NaCl or ABTGC supplied with 5 μM SNP, respectively, and monitored for their pyoverdine fluorescence by using a Tecan Infinite Pro2000 microplate reader. Means and s.d. in relative fluorescence units (RFU) from triplicate experiments are shown. ( d ) Reversion of yhjH- dispersed cells in ABTGC, 0.9% NaCl and ABTGC supplied with 0.25% arabinose. YhjH -dispersed cells were inoculated into microplates containing ABTGC, 0.9% NaCl or ABTGC supplied with 0.25% arabinose, respectively, and monitored for their pyoverdine fluorescence using a Tecan Infinite Pro2000 microplate reader. Means and s.d. in RFU from triplicate experiments are shown. ( e ) Expression of the p pvdA -gfp fusion in planktonic cells and dispersed cells after 5-h dispersal. Representative confocal images are shown for each condition. Scale bars, 10 μm. Full size image Dispersed cells have unique physiology To characterize and compare the gene expression profile of chemically and enzymatically dispersed cells (SNP exposure versus yhjH PDE induction) with those of planktonic and biofilm cells, we performed transcriptomic analysis. The heatmap of the genes that were differently expressed among planktonic P. aeruginosa cells, biofilm cells and dispersed cells is illustrated in Fig. 2a . Further examination of the transcriptome by principal component analysis revealed that the dispersed cells have a distinct physiology compared with both planktonic and biofilm cells ( Fig. 2b ). Planktonic cells exhibit a higher expression level of the genes involved in las and rhl quorum sensing (for example, lasA , lasR , rhlA , rhlB , rhlR ) compared with biofilm and dispersed cells ( Supplementary Data 1 ). Biofilm cells exhibit a higher expression level of the genes involved in matrix protein synthesis (for example, cdrA , cdrB ) and a lower expression level of the genes involved in motility and chemotaxis (for example, pilA , fliC , aer ) compared with planktonic and dispersed cells ( Supplementary Data 1 ). Dispersed cells exhibit a higher expression level of the genes involved in virulence (for example, secB ) and a lower expression level of the genes involved in iron uptake (for example, pvdA , pvdS ) compared with planktonic cells and biofilm cells ( Supplementary Data 1 ). 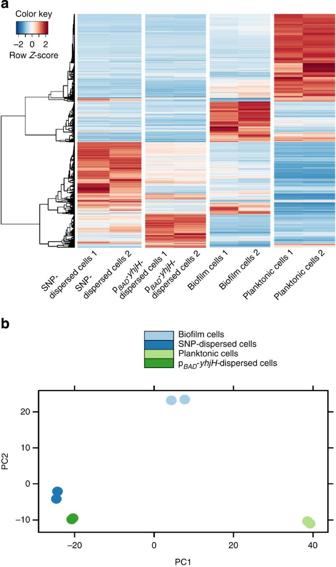Figure 2: Gene expression analysis of dispersed cells. Hierarchical clustering analysis and a heatmap of the differentially expressed genes ofP. aeruginosaplanktonic cells, SNP-dispersed cells,yhjH-dispersed cells and biofilm cells are shown ina. PCA of gene expression ofP. aeruginosaplanktonic cells, SNP-dispersed cells,yhjH-dispersed cells and biofilm cells is shown inb. Raw data of RNA-Seq were normalized using the DESeq package before clustering analysis and PCA analysis. Red: Higher expression levels; blue: lower expression levels. The differentially expressed genes (fold-change >5, adjustedP-value <0.05) between any pairs of (i) SNP-dispersed cells, (ii)yhjH-dispersed cells, (iii) planktonic cells and (iv) biofilm cells were identified by performing a negative binomial test using the DESeq package of R/Bioconductor. The full list of genes that were differentially expressed between any pairs of the above four groups is provided inSupplementary Data 1. Figure 2: Gene expression analysis of dispersed cells. Hierarchical clustering analysis and a heatmap of the differentially expressed genes of P. aeruginosa planktonic cells, SNP-dispersed cells, yhjH -dispersed cells and biofilm cells are shown in a . PCA of gene expression of P. aeruginosa planktonic cells, SNP-dispersed cells, yhjH -dispersed cells and biofilm cells is shown in b . Raw data of RNA-Seq were normalized using the DESeq package before clustering analysis and PCA analysis. Red: Higher expression levels; blue: lower expression levels. The differentially expressed genes (fold-change >5, adjusted P -value <0.05) between any pairs of (i) SNP-dispersed cells, (ii) yhjH -dispersed cells, (iii) planktonic cells and (iv) biofilm cells were identified by performing a negative binomial test using the DESeq package of R/Bioconductor. The full list of genes that were differentially expressed between any pairs of the above four groups is provided in Supplementary Data 1 . Full size image Using a negative binomial test with a P -value cut-off of 0.05 and a fold-change cut-off of 5, we found that 353 genes ( Supplementary Data 1 ) were upregulated and 280 genes ( Supplementary Data 1 ) were downregulated in both dispersal conditions compared with planktonic cells. While the SNP-dispersed cells and yhjH -dispersed cells were generally similar to each other, a few differences in gene expression remained between these types of dispersed cells ( Fig. 2 ). We showed that dispersed cells are in a distinct stage in the transition from biofilm to planktonic lifestyle, as supported by the evidence showing that biofilm cells differ from dispersed cells [15] . We identified multiple T2SS genes, such as PA3820 ( secF ) and PA3821 ( secD ), that were at least fivefold upregulated in dispersed cells compared with planktonic cells. Hence, we hypothesized that dispersed cells might be enhanced in virulence. Low expression levels of small RNAs in dispersed cells The expression level of the small non-coding RNA RsmY was lower in biofilm-dispersed cells ( Supplementary Data 1 ) compared with planktonic cells, and we further found that biofilm-dispersed cells had a low expression of both rsmY and rsmZ , according to reporter fusion measurements ( Fig. 3a ). These low expression levels of rsmY and rsmZ were consistent with the important roles of these two non-coding RNAs in regulating biofilm formation [22] , type III secretion [22] , iron siderophore synthesis [23] , motility [22] and quorum sensing [24] . We further used qRT–PCR to measure the expression levels of two of the RsmYZ-regulated genes, secD [25] and pvdS [23] . Consistent with our RNA-seq analysis, qPCR showed that the secD gene is upregulated and that the pvdS gene is downregulated in dispersed cells compared with planktonic cells ( Fig. 3b ). 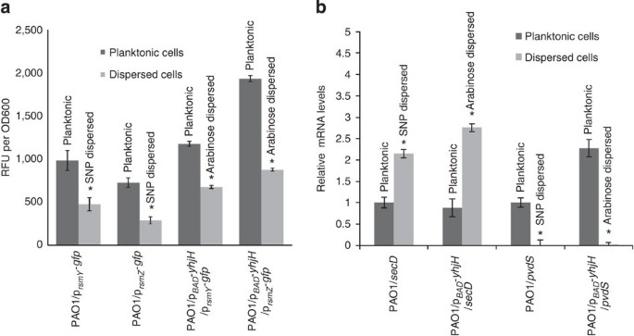Figure 3: The physiological markers of dispersed cells. (a) Expression ofrsmY-gfpandrsmZ-gfpinP. aeruginosaplanktonic cells, SNP-dispersed cells,yhjH-dispersed cells. (b) Expression ofsecDandpvdSmessenger RNA inP. aeruginosaplanktonic cells, SNP-dispersed cells andyhjH-dispersed cells. Means and s.d. in relative fluorescence units (RFU) from triplicate experiments are shown. Student’st-test was performed for testing differences between groups. *P<0.01. Figure 3: The physiological markers of dispersed cells. ( a ) Expression of rsmY-gfp and rsmZ-gfp in P. aeruginosa planktonic cells, SNP-dispersed cells, yhjH -dispersed cells. ( b ) Expression of secD and pvdS messenger RNA in P. aeruginosa planktonic cells, SNP-dispersed cells and yhjH -dispersed cells. Means and s.d. in relative fluorescence units (RFU) from triplicate experiments are shown. Student’s t -test was performed for testing differences between groups. * P <0.01. Full size image Virulence of dispersed cells in vitro The acute infections caused by P. aeruginosa are usually invasive, and its pathogenicity is attributed to the secretion of exotoxins and proteases via different classes of secretion systems. The T3SS components, including Psc, are important in the formation of the injectosome and in establishing extracellular association with host cells [26] . Alveolar macrophages are important in the defence against P. aeruginosa invasion in the human lungs because they prevent acute pneumonia and later chronic infections [27] , [28] . The effective phagocytosis of pathogens is highly important in preventing their dissemination throughout the host. RsmY and RsmZ are known to negatively regulate type III secretion in P. aeruginosa by antagonizing RsmA, a posttranscriptional regulator [29] , [30] . A Δ rsmY Δ rsmZ double mutant has a higher level of type III secretion and is more virulent than single Δ rsmY or Δ rsmZ mutants [31] . Because the expressions of both rsmY and rsmZ were lower in dispersed cells than they were in planktonic cells, we hypothesized that dispersed cells could activate their type III secretion and thus be more virulent to macrophages than planktonic cells. As expected, the internalization of biofilm-dispersed cells by macrophages was nearly 100-fold less efficient than that of planktonic cells after 2 h of co-infection with macrophages ( Fig. 4a ), highlighting the capacity of dispersed cells to resist phagocytosis. Moreover, dispersed cells were able to kill macrophages at a higher rate than planktonic cells ( Fig. 4b ). A higher proportion of macrophages were stained with the ‘dead cell stain’ propidium iodide (PI) after 2 h of co-infection followed by 2 h incubation with dispersed cells, indicating that dispersed bacteria exhibit a significantly higher level of cytotoxicity compared with the planktonic bacteria. We used a Δ pscJ mutant in our virulence assays to demonstrate that T3SS is essential for eliciting a virulent response in dispersed cells. The role of pscJ in the translocation of exotoxins such as ExoT to the host cells has been well documented [32] . The mutagenesis of pscJ results in the reduced secretion of exotoxins. We confirmed that the inactivation of pscJ led to both the attenuated evasiveness and cytotoxicity of dispersed cells against macrophages at similar levels to planktonic cells ( Fig. 4c,d ). 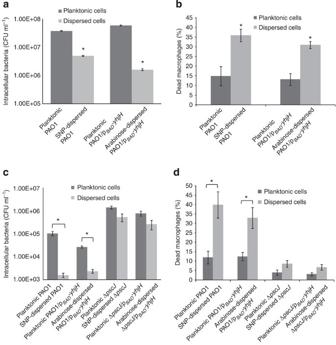Figure 4: Phagocytosis evasion (a,c) and macrophage killing (b,d) by planktonic cells, SNP-dispersed cells andyhjH-dispersed cells fromP. aeruginosaPAO1 and the ΔpscJmutant. Fora,c, the means and s.d. from triplicate experiments of CFU are shown. Student’st-test was performed to test differences between groups.*P<0.01. Forb,d, the means and s.d. ratio of dead cells over live cells enumerated from five images are shown. Student’st-test was performed to test differences between groups.*P<0.01. Note: TheP. aeruginosastrains forc,dare from the PAO1alineage (details described in Methods). Figure 4: Phagocytosis evasion ( a , c ) and macrophage killing ( b , d ) by planktonic cells, SNP-dispersed cells and yhjH -dispersed cells from P. aeruginosa PAO1 and the Δ pscJ mutant. For a , c , the means and s.d. from triplicate experiments of CFU are shown. Student’s t -test was performed to test differences between groups. * P <0.01. For b , d , the means and s.d. ratio of dead cells over live cells enumerated from five images are shown. Student’s t -test was performed to test differences between groups. * P <0.01. Note: The P. aeruginosa strains for c , d are from the PAO1 a lineage (details described in Methods). Full size image Virulence of dispersed cells in vivo C. elegans is an important model for studying host–pathogen interactions because the virulence factors identified using the nematode host can also be relevant to mammalian hosts [33] . The C. elegans liquid killing assay revealed that dispersed cells were more virulent than planktonic cells because they were able to kill up to 90% of the nematodes after 6 h of feeding, compared with the 40% of total worms killed by planktonic cells ( Fig. 5a ). The involvement of the induction of secretion systems in the enhancement of virulence in dispersed P. aeruginosa cells was also examined. We found that type II secretion is essential for C. elegans killing because a Δ secB mutant is severely hampered in its ability to rapidly kill C. elegans ( Fig. 5b ). We noted that the SNP-dispersed Δ secB cells were more virulent than the planktonic Δ secB cells and were able to kill C. elegans less efficiently than SNP-dispersed PAO1 ( Fig. 5 ), possibly because the addition of SNP slightly increases the growth rate of P. aeruginosa . These results indicated that biofilm-dispersed cells are more virulent than planktonic cells with respect to acute infections. 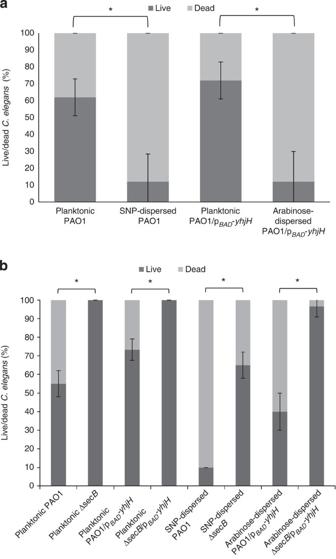Figure 5:C. elegansliquid killing by planktonic cells, SNP-dispersed cells andyhjH-dispersed cells fromP. aeruginosaPAO1 (a) and ΔsecBmutant (b). Means and s.d. from triplicate experiments are shown. Student’st-test was performed to test differences between groups. *P<0.01. Note: TheP. aeruginosastrains forbare from the PAO1alineage (details described in Methods). Figure 5: C. elegans liquid killing by planktonic cells, SNP-dispersed cells and yhjH -dispersed cells from P. aeruginosa PAO1 ( a ) and Δ secB mutant ( b ). Means and s.d. from triplicate experiments are shown. Student’s t -test was performed to test differences between groups. * P <0.01. Note: The P. aeruginosa strains for b are from the PAO1 a lineage (details described in Methods). Full size image Dispersed cells are highly sensitive to iron stress While biofilms create confined areas of persistent infections, dispersed cells are instrumental in the spreading and subsequent transmission of diseases [34] , [35] , [36] . With the strong implication that freshly dispersed cells are highly virulent to the host cells, it is important to identify their potential weaknesses. Such knowledge is important for the development of containment and eradication principles. Our transcriptomic analysis showed that biofilm dispersal caused the downregulation of genes related to the synthesis of the major iron siderophore pyoverdine and other iron uptake systems. Siderophores are produced by many bacterial species to scavenge iron from the environment. In P. aeruginosa , the pvd and pch operons are involved in the production of pyoverdine and pyochelin, respectively [37] . Our transcriptomic analysis showed that the expression of the iron starvation sigma factor, pvdS [38] , was downregulated in both types of dispersed cells compared with planktonic cells ( Supplementary Data 1 ). In accordance, the expression of other PvdS-regulated genes, such as pvdG , pvdH , pchB , pchC , pchD , pchE , pchG , pchF and fpvA , were all downregulated in biofilm-dispersed cells compared with planktonic cells. The expression level of a P pvdA - gfp transcriptional fusion in dispersed cells was significantly lower than that in planktonic cells ( Fig. 6a ). This correlated with the finding that the production of pyoverdine in dispersed cells is lower than that in planktonic cells ( Fig. 6b ). A difference in growth in the presence of 160 μg ml −1 of the 2,2′-dipyridyl (DIPY) iron chelator demonstrated that dispersed cells were more susceptible to iron stress than planktonic cells ( Fig. 6c,d ). 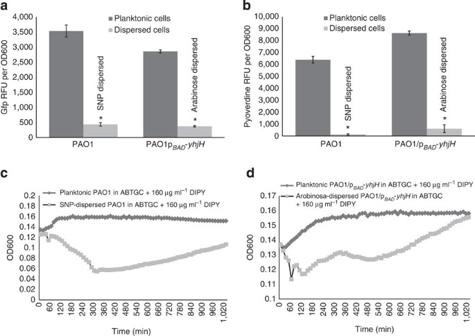Figure 6: Pyoverdine synthesis and iron chelator tolerance assays forP. aeruginosaPAO1 planktonic cells, SNP-dispersed cells andyhjH-dispersed cells. Expression of the ppvdA-gfptranscriptional fusion (a) and production of pyoverdine (b) were measured in 96-well microplates. The pyoverdine fluorescence levels (excitation wavelength, 400 nm; emission wavelength, 450 nm) of supernatants ofP. aeruginosaovernight cultures were recorded using the Tecan Infinite Pro2000 microplate reader. Means and s.d. in relative fluorescence units from triplicate experiments are shown fora,b. Student’st-test was performed to test differences between groups. *P<0.01. Growth of planktonic and SNP-dispersed cells (c), planktonic andyhjH-dispersed cells (d) in the presence of 160 μg ml−1of the iron chelator DIPY were monitored in 96-well microplates. Means from triplicate experiments are shown forc,d. Figure 6: Pyoverdine synthesis and iron chelator tolerance assays for P. aeruginosa PAO1 planktonic cells, SNP-dispersed cells and yhjH -dispersed cells. Expression of the p pvdA - gfp transcriptional fusion ( a ) and production of pyoverdine ( b ) were measured in 96-well microplates. The pyoverdine fluorescence levels (excitation wavelength, 400 nm; emission wavelength, 450 nm) of supernatants of P. aeruginosa overnight cultures were recorded using the Tecan Infinite Pro2000 microplate reader. Means and s.d. in relative fluorescence units from triplicate experiments are shown for a , b . Student’s t -test was performed to test differences between groups. * P <0.01. Growth of planktonic and SNP-dispersed cells ( c ), planktonic and yhjH -dispersed cells ( d ) in the presence of 160 μg ml −1 of the iron chelator DIPY were monitored in 96-well microplates. Means from triplicate experiments are shown for c , d . Full size image Iron chelator reduces the survival of dispersed cells While many studies focus on the chemical induction of dispersal as an anti-biofilm strategy, little attention has been paid to the cells that are liberated from the biofilms. Because these cells show an increased ability to avoid macrophage-mediated phagocytosis, dispersing agents are likely to be administered in combination with other antimicrobials that would limit the growth and the spread of dispersed cells. The combined administration of a biofilm-dispersing agent such as SNP with an iron chelator to mature (72 h) P. aeruginosa biofilms resulted in dispersing agents efficiently dispersing biofilms ( Figs 7 , 8 ). The addition of 100 μg ml −1 DIPY reduced the viability of the dispersed cells significantly ( Figs 7 , 8 ). Furthermore, we showed that applying 10 μg ml −1 tobramycin together with dispersing agents and an iron chelator almost completely eradicated the biofilms ( Figs 7 , 8 ). 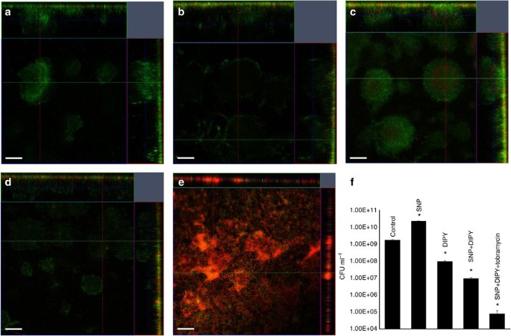Figure 7: Synergistic effect of a dispersing agent and an iron chelator on mature biofilms. Here, 72-h biofilms of GFP-tagged PAO1 grown in ABTG medium were treated as follows: no treatment (medium control) (a), dispersing agent SNP (b), iron chelator DIPY (c), combination of SNP and DIPY (d) and combination of SNP, DIPY and tobramycin (e) for 24 h, after which they were stained with PI and images were acquired by confocal laser scanning microscope. Representative image from triplicate experiments is shown for each condition. Live cells appear green, and dead cells appear yellow or red. The central pictures show horizontal optical sections, and the flanking pictures show vertical optical sections. Scale bars, 20 μm. The dispersed cells were collected from the flow chamber effluent after treatments were grown on LB agar plates overnight at 37 °C. Colonies were enumerated, and colony-forming units ml−1(CFU ml−1) were calculated (f). Means from triplicate experiments are shown forf. Student’st-test was performed to test differences between groups. *P<0.01. Figure 7: Synergistic effect of a dispersing agent and an iron chelator on mature biofilms. Here, 72-h biofilms of GFP-tagged PAO1 grown in ABTG medium were treated as follows: no treatment (medium control) ( a ), dispersing agent SNP ( b ), iron chelator DIPY ( c ), combination of SNP and DIPY ( d ) and combination of SNP, DIPY and tobramycin ( e ) for 24 h, after which they were stained with PI and images were acquired by confocal laser scanning microscope. Representative image from triplicate experiments is shown for each condition. Live cells appear green, and dead cells appear yellow or red. The central pictures show horizontal optical sections, and the flanking pictures show vertical optical sections. Scale bars, 20 μm. The dispersed cells were collected from the flow chamber effluent after treatments were grown on LB agar plates overnight at 37 °C. Colonies were enumerated, and colony-forming units ml −1 (CFU ml −1 ) were calculated ( f ). Means from triplicate experiments are shown for f . Student’s t -test was performed to test differences between groups. * P <0.01. 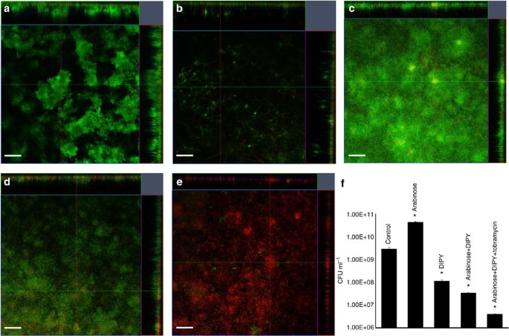Figure 8: Synergistic effect ofyhjH-mediated dispersal and an iron chelator on mature biofilms. Here, 72 h biofilms of GFP-tagged PAO1/pBAD-yhjHgrown in ABTG medium were treated medium control (a), arabinose (b), iron chelator DIPY (c), combination of arabinose and DIPY (d) and a combination of arabinose, DIPY and tobramycin (e) for 24 h, after which they were stained with PI and images were acquired by confocal laser scanning microscope. A representative image from triplicated experiments is shown for each condition. Live cells appear green, and dead cells appear yellow or red. The central pictures show horizontal optical sections, and the flanking pictures show vertical optical sections. Scale bars, 20 μm. The dispersed cells were collected from the flow chamber effluent after treatments grown on LB agar plates overnight at 37 °C. Colonies grown were enumerated, and colony-forming units ml−1(CFU ml−1) were calculated (f). Means from triplicate experiments are shown forf. Student’st-test was performed to test differences between groups. *P<0.01. Full size image Figure 8: Synergistic effect of yhjH -mediated dispersal and an iron chelator on mature biofilms. Here, 72 h biofilms of GFP-tagged PAO1/p BAD - yhjH grown in ABTG medium were treated medium control ( a ), arabinose ( b ), iron chelator DIPY ( c ), combination of arabinose and DIPY ( d ) and a combination of arabinose, DIPY and tobramycin ( e ) for 24 h, after which they were stained with PI and images were acquired by confocal laser scanning microscope. A representative image from triplicated experiments is shown for each condition. Live cells appear green, and dead cells appear yellow or red. The central pictures show horizontal optical sections, and the flanking pictures show vertical optical sections. Scale bars, 20 μm. The dispersed cells were collected from the flow chamber effluent after treatments grown on LB agar plates overnight at 37 °C. Colonies grown were enumerated, and colony-forming units ml −1 (CFU ml −1 ) were calculated ( f ). Means from triplicate experiments are shown for f . Student’s t -test was performed to test differences between groups. * P <0.01. Full size image The present study suggests that cells from programmed biofilm dispersal belong to an important and unique intermediate phase in the biphasic life cycle of bacteria. C-di-GMP-mediated dispersal represents one of the best characterized programmed biofilm dispersal processes. The dispersed cells have a low intracellular c-di-GMP content compared with biofilm cells and will eventually become motile and fast growing ( Fig. 1 ). Hence, the dispersed cells were, until now, thought to be similar to planktonic cells and assumed to be easily eradicated by the host immune system and antimicrobials [6] . While the major advantage of dispersal is to allow the dissemination of a species to a larger range of environments, there is no doubt that dispersed cells face various environmental stresses, including predation. In this communication, we monitored the dynamics of biofilm dispersal induced by lowering the c-di-GMP content in the bacteria using both chemical and enzymatic approaches. There was a 2-h transient period in which dispersed cells kept their phenotypes, even without the presence of dispersal agents ( Fig. 1 ). The dispersed cells retained their phenotypes for a longer duration when there were no proper growth conditions ( Fig. 1 ). The growth of dispersed cells in fresh medium likely leads to the synthesis of c-di-GMP, thus reverting them to normal planktonic cells. The growth of dispersed cells in the presence of dispersal agents constitutively activates PDEs and keeps the c-di-GMP content low, resulting in dispersed cells being unable to revert to planktonic cells ( Fig. 1 ). It is likely that dispersed cells will be able to disseminate within a host while maintaining their specific dispersed cell phenotype if future biofilm-dispersing drugs are used clinically. We further elaborated on our previous analysis of dispersed cells, which showed an induction of genes conferring resistance towards antimicrobial peptides in the dispersed cells [19] . Our data support a model in which dispersed cells display a number of unique phenotypes ( Fig. 1 ). The unique phenotype of dispersed cells might result from the distinct physiology of biofilm cells and the rapid reduction of the intracellular c-di-GMP content via dispersing agents. In contrast, the treatment of planktonic cells with the dispersal agents only slightly reduced their pyoverdine expression ( Supplementary Fig. 1 ). Interestingly, this study showed that biofilm-dispersed cells, in contrast to their planktonic counterparts, are characterized by lower levels of the regulatory small RNAs RsmY and RsmZ ( Fig. 3 ). Recently, RsmY and RsmZ were found to positively regulate iron siderophore production in P. aeruginosa [23] . In addition, the Gac/Rsm system was shown to negatively affect the intracellular c-di-GMP content [22] . The present study shows that the biofilm-dispersed cells not only have a lower intracellular c-di-GMP content than planktonic cells but also have a lower expression level of rsmY and rsmZ compared with planktonic cells, which in turn reduces siderophore production ( Supplementary Data 1 ). Here, we show that dispersed cells are more virulent against immune cells and C. elegans than their planktonic counterparts. The T3SS psc gene is essential in eliciting full virulence against macrophages by dispersed cells ( Fig. 4 ). The virulence of dispersed cells might contribute to the notorious difficulty of treating chronic infections. We also show that the T2SS is induced in dispersed cells and is required for the rapid killing of C. elegans by dispersed cells ( Fig. 5 ). A recent study showed that the GacS/GacA system, which is known to positively regulate rsmY and rsmZ expression, negatively regulates the T2SS of P. aeruginosa M18 (ref. 25 ). The dispersed cell physiology is, to a certain extent, similar to that of early exponential phase cells, which also have lower expression levels of rsmY and rsmZ and higher expression levels of type II and type III secretion systems compared with late exponential phase cells [39] , [40] . However, the early exponential phase of growth can only be reached by cultivating planktonic bacterial cells under optimal growth conditions for several generations, while the dispersed cell phenotype appeared immediately after dispersal from biofilms and can be retained without growth ( Fig. 1 ). Taken together with the present study, these data strongly suggest that the process of dispersal confers ‘protection-in-advance mechanisms’ to cope with environmental insults. In our proposed, modified model of the biofilm life cycle, we place dispersed cells as a unique intermediate step between the planktonic and the biofilm lifestyles ( Fig. 9 ). 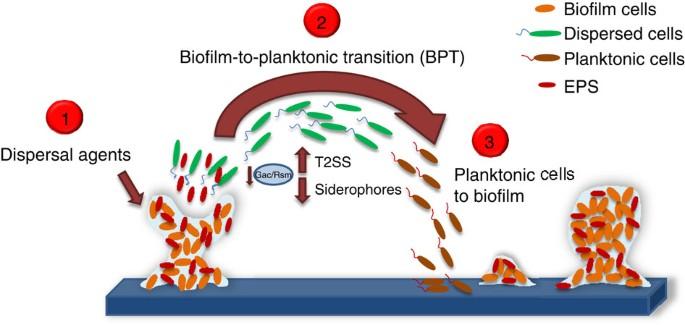Figure 9: A model of the biofilm–planktonic life cycle, with dispersed cells as a unique intermediate between planktonic and biofilm lifestyles. (1) The addition of dispersal agents can cause biofilm dispersal and release dispersed cells (shown in green). (2) Dispersed cells have lower expression levels of the Gac-dependent small RNAs RsmY and RsmZ, higher expression of T2SS and lower production of siderophores such as pyoverdine compared with planktonic cells (shown in brown). (3) Dispersed cells revert to the planktonic mode, which eventually colonize new surfaces and form biofilms. Figure 9: A model of the biofilm–planktonic life cycle, with dispersed cells as a unique intermediate between planktonic and biofilm lifestyles. (1) The addition of dispersal agents can cause biofilm dispersal and release dispersed cells (shown in green). (2) Dispersed cells have lower expression levels of the Gac-dependent small RNAs RsmY and RsmZ, higher expression of T2SS and lower production of siderophores such as pyoverdine compared with planktonic cells (shown in brown). (3) Dispersed cells revert to the planktonic mode, which eventually colonize new surfaces and form biofilms. Full size image In a bid to eradicate biofilm infections, Christensen et al. [41] recently proved that the manipulation of the intracellular c-di-GMP content is able to cause biofilm dispersal in an implant-based mouse infection model. While this previous study showed an in vivo proof of concept of biofilm dispersal, it raised the question of the safety of releasing highly virulent dispersed cells, which can potentially result in the spread of infections or septic shock. In addition to the SNP and yhjH -induced biofilm dispersal, macrophage treatment can induce biofilm dispersal, and the dispersed cells showed similar phenotypes to the SNP and yhjH -dispersed cells ( Supplementary Fig. 2 ). Studies on dispersed cells from Group A Streptococcus (ref. 34 ) and Streptococcus pneumonia (ref. 35 ) in murine models and enteropathogenic E. coli in human volunteers [36] demonstrated increased disease progression; these findings support our data that dispersed cells are highly virulent and can be involved in heightening disease severity. The ability of dispersed cells to maintain their dispersed state for hours before reverting back to the planktonic mode also implies that they can remain highly virulent within the host before re-colonizing a new infection site. Thus, potential biofilm dispersal strategies should be combined with antimicrobial strategies that are capable of eliminating dispersed cells. A thorough understanding of the physiology of biofilm-dispersed cells will be important for devising combinatory therapies that aim at biofilm dissolution. We found that dispersed cells have a lower production of iron siderophores such as pyoverdine than do planktonic cells. Although pyoverdine is an important siderophore in bacterial growth [42] , it appears that siderophores are not required in dispersed cells. This will subject the dispersed cells to continual iron stress. In agreement with this hypothesis, the addition of the iron chelator DIPY inhibited the growth of freshly dispersed cells. Lactoferrin produced by the innate immune system can sequester iron [43] and might play a role in reducing the spread of dispersed cells to new infection sites. We envision that synergistic treatments of biofilms with dispersing agents and DIPY in combination with conventional antibiotics such as colistin (which kills non-growing cells) and ciprofloxacin (which kills growing cells) will reduce local chronic infections and reduce the spread of highly virulent dispersed cells into systemic circulation in the host. Bacterial strains and growth conditions The bacterial strains, plasmids and primers used in this study are listed in Table 1 . E. coli DH5a strain was used for standard DNA manipulations. LB medium was used to cultivate E. coli strains. Batch cultivation of P. aeruginosa strains was carried out at 37 °C in ABTG (ABT minimal medium [44] supplemented with 5 g glucose l −1 ) or ABTGC (ABT minimal medium supplemented with 2 g glucose l −1 and 2 g casamino acids l −1 ). For plasmid maintenance in E. coli , the medium was supplemented with 100 μg ampicillin (Ap) ml −1 , 15 μg gentamicin (Gm) ml −1 , 15 μg tetracycline (Tc) ml −1 or 8 μg chloramphenicol ml −1 . For marker selection in P. aeruginosa , 30 μg Gm ml −1 , 50 μg Tc ml −1 or 200 μg carbenicillin ml −1 were used, as appropriate. Table 1 Bacterial strains and plasmids used in this study. Full size table Generation of planktonic, biofilm and dispersed cells A microplate biofilm formation assay was first carried out in ABTGC medium as previously described [19] . A cell scraper (Nunc, Roskilde, Denmark) was used to scrape the biofilms from the surface of 24-well plates (Nunc). To generate dispersed cells, the biofilms were washed three times with 0.9% NaCl and resuspended in ABTGC medium containing 5 μM nitric oxide donor SNP dihydrate for PAO1 biofilms or 0.25% arabinose for PAO1/p BAD - yhjH biofilms. Biofilms were dispersed at 37 °C for 5 h without shaking until collection. Colony-forming units (CFU) of dispersed and planktonic cells were monitored throughout the dispersal process by serial dilution in 0.9% NaCl and plating on LB agar plates. Planktonic PAO1 cells were cultivated in ABTGC medium at 37 °C with shaking for same period as the biofilm dispersal procedure until they reached late exponential/early stationary phase. Experiments were performed in triplicate, and the results are shown as the mean±s.d. Measurement of the stability of dispersed cells Planktonic and dispersed cells were generated as described above and adjusted to OD 600 =0.15 in ABTGC and in 0.9% NaCl with and without the presence of dispersal agents. The cells were then incubated in 96-well plates (Nunc) at 37 °C. Pyoverdine fluorescence (excitation maximum 400 nm, emission maximum 450 nm) and OD 600 were recorded by the microplate reader (Tecan Infinite 2000) every 15 min. Experiments were performed in triplicate, and the results are shown as the mean±s.d. To examine the population homogeneity of the dispersed cells, a PAO1/p pvdA - gfp strain that was tagged with the pyoverdine synthesis report gene fusion, p pvdA - gfp was used in the dispersal experiments. Dispersed PAO1/p pvdA - gfp cells after 5 h of induction were observed under confocal laser scanning microscope. Experiments were performed in triplicate, and representative images of each condition are shown in the results. C-di-GMP quantification Planktonic and dispersed cells were generated as described above. Cells were washed three times with 1 mM ice cold ammonium acetate and resuspended in ice cold buffer (40% acetonitrile, 40% methanol and 20% ddH 2 O). The cells were lysed using a probe ultrasonicator (Sonics SM VibraCell CVX750). Cell debris was removed by ultracentrifugation, leaving behind the supernatant containing metabolites and c-di-GMP. Samples were concentrated by a vacuum concentrator (SpeedVac) and resuspended in 100 μl per 1 mM ammonium acetate. Each sample was loaded into a vial for high-performance liquid chromatography (Agilent, USA) analysis, with a detection wavelength of 254 nm to measure the c-di-GMP concentration [45] . A C18 column (Ascentis) was used with 95% solvent A (0.9% NaCl) and 5% solvent B (100% acetonitrile), at a flow rate of 0.5 ml min −1 . The c-di-GMP concentration was normalized by total protein concentration. The relative c-di-GMP concentrations of dispersed cells against planktonic cells are shown. Experiments were performed in triplicate, and the results are shown as the mean±s.d. RNA preparation Bacterial cells were collected as described above. Total RNA was extracted with an RNeasy Protect Bacteria Mini Kit with on-column DNase digestion (Qiagen). A Turbo DNA-free vigorous protocol was used for a second round of DNase treatment (Ambion). The integrity of the total RNA and the level of DNA contamination were assessed with an Agilent 2100 Bioanalyzer (Agilent Technologies) and Qubit 2.0 Fluorometer (Invitrogen). 16S, 23S and 5S rRNA were removed using the Ribo-Zero Magnetic Kit (Bacteria) (Epicentre). RNA sequencing and data analysis Gene expression analysis was conducted via Illumina RNA sequencing (RNA-Seq technology). RNA-Seq was conducted for two biological replicates of each sample. Libraries were produced using an Illumina TruSeq Stranded messenger RNA Sample Prep Kit. The libraries were sequenced using the Illumina MiSeq V2 platform with a paired-end protocol and read lengths of 150 nt. The sequence reads were mapped onto the P. aeruginosa PAO1 reference genome, which is available for download from the Pseudomonas Genome Database (http://www.pseudomonas.com) [46] , using the ‘RNA-Seq and expression analysis’ application of the CLC genomics Workbench 6.0 (CLC Bio, Aarhus, Denmark). The following criteria were used to filter the unique sequence reads: maximum number of hits for a read of 1, minimum length fraction of 0.9, minimum similarity fraction of 0.8 and maximum number of two mismatches. A constant of 1 was added to the raw transcript count value to avoid any problems caused by 0. The transcript count table was subjected to the DESeq package [47] of R/Bioconductor [48] for statistical analysis. The transcript counts were normalized to the effective library size. The differentially expressed genes were identified by performing a negative binomial test. Transcripts were stringently determined as differentially expressed when they had a fold-change larger than five and an adjusted P -value smaller than 0.05. Hierarchical clustering analysis was performed, and a heatmap was drawn for the differentially expressed genes between any pairs of the following: (i) SNP-dispersed cells, (ii) yhjH -dispersed cells, (iii) planktonic cells and (iv) biofilm cells, using the heatmap.2 package of R/Bioconductor [48] . Furthermore, the normalized counts were stabilized according to their variance as outlined in the DESeq package tutorial, and a principle component analysis plot was generated. qRT–PCR analysis Total RNA was extracted using RNeasy Mini Kit (Qiagen) with on-column DNase digestion. The purity and concentration of the RNA were determined by NanoDrop spectrophotometry, and the integrity of RNA was measured using an Agilent 2200 TapeStation System. The elimination of contaminating DNA was confirmed via the real-time PCR amplification of the rpoD gene using total RNA as the template. Quantitative reverse transcriptase PCR (qRT–PCR) was performed using a two-step method. First-strand cDNA was synthesized from total RNA using SuperScript III First-Strand Synthesis SuperMix kit (Cat. No. 18080-400, Invitrogen). The cDNA was used as a template for qRT–PCR with a SYBR Select Master Mix kit (Cat. No. 4472953, Applied Biosystems by Life Technologies) on an Applied Biosystems StepOnePlus Real-Time PCR System. The gene rpoD was used as an endogenous control. Melting curve analyses were employed to verify the specific single-product amplification. Construction of the transcriptional fusions The rsmZ-gfpmut3b* and rsmY-gfpmut3b*- based monitor plasmids pRV59_1 and pRV60_1 were constructed by subcloning the rsmZ and rsmY promoter regions of pMP220 rsmZ-lacZ and pMP220 rsmY-lacZ (ref. 49 ) into pMH305 (ref. 50) [50] , a pUCP22NotI-based expression vector carrying a promoterless gfpmut3b* gene (pMH305 carries the RBSII- gfp (Mut3)-T 0 -T 1 fragment of pJBA25 (ref. 51) [51] in the NotI site). The promoter regions were excised by digestion with KpnI and EcoRI and inserted into KnpI / EcoRI -digested pMH305, thereby generating the p rsmZ -gfpmut3b* and p rsmY -gfpmut3b* transcriptional fusions. The ligation mixtures were transformed into E. coli K-12 and distinguished using selective plates containing 100 μg ampicillin ml −1 . The plasmid constructs were verified by restriction analysis and subsequently moved into P. aeruginosa by electroporation and plating on 30 μg Gm ml −1 (ref. 52 ). p rsmY -gfp and the p rsmZ -gfp reporter assay Planktonic and biofilm-dispersed P. aeruginosa strains containing p rsmY -gfp and the p rsmZ -gfp biosensors were cultivated in 37 °C, as described above. A total of 200 μl of cultures were transferred into each of the wells of a 96-well microplate. The expression of p rsmY -gfp and p rsmZ -gfp in P. aeruginosa was measured using a microplate reader (Tecan Infinite 2000). OD 600 and Gfp fluorescence readings (expressed in relative fluorescence units) were recorded for each well of the 96-well microplate. Experiments were performed in triplicate, and the results are shown as the mean±s.d. Cell culturing experiments The permanent mouse macrophages cell line RAW264.7 (ATCC No. TIB-71) was cultured in Dulbecco’s modified Eagle’s medium (DMEM) (Life Technologies), supplemented with 10% fetal bovine serum (Gibco). Cells were incubated in 25 cm 2 cell culture flasks at a density of 1.0 × 10 6 cells ml −1 at 37 °C and 5% CO 2 for 72 h. Macrophage phagocytosis assay Here, 5 × 10 5 RAW264.7 macrophages were grown in 24-well culture plates. Triplicate cultures were infected with planktonic or dispersed bacteria suspension at a multiplicity of infections of 100:1. The co-cultures were incubated for 2 h at 37 °C and 5% CO 2 . More than 90% of the macrophage cells remained live after 2 h co-culture. To remove extracellular bacteria, the macrophages were washed with phosphate-buffered saline three times. Infected macrophages were then lysed with ddH 2 O containing 0.5% Triton X-100 (ref. 53 ). The cell lysates were then serially diluted, and 100 μl of each dilution was plated on triplicate LB agar plates and incubated at 37 °C overnight. The number of colonies was enumerated, and CFU ml −1 were tabulated. Experiments were performed in triplicate, and the results are shown as the mean±s.d. Cytotoxicity assay for macrophages Here, 5 × 10 5 RAW264.7 macrophages were grown in 24-well culture plates. Triplicate cultures were infected with planktonic or dispersed bacteria suspensions at a multiplicity of infections of 100:1. The co-cultures were incubated for 2 h at 37 °C and 5% CO 2 . Extracellular cells were washed away three times with phosphate-buffered saline, and macrophages were incubated for a further 2 h in fresh DMEM. The cytotoxicity of the engulfed bacteria (either planktonic or dispersed) was determined by monitoring cell integrity with PI, which only enters cells that are dead. Cells that stained red under the epifluorescent microscopy (Zeiss) were counted as dead. The ratio of dead cells to live cells, as enumerated from five images, was then calculated and averaged. Experiments were performed in triplicates, and the results are shown as the mean±s.d. Macrophage–biofilm interaction assay Sterile glass coverslips were used for biofilm formation; they were immersed vertically in 50 ml conical centrifuge tubes (Falcon, Fisher Scientific) filled with 10 ml ABTGC medium with an initial inoculum of 10 6 cells ml −1 gfp-tagged P. aeruginosa PAO1 strain, as previously described [54] . Coverslips were removed from conical tubes after 24 h incubation at 37 °C and submerged in 0.9% NaCl to wash off unattached cells or aggregates, leaving behind only biofilms. Then, 5 × 10 5 macrophages ml −1 in DMEM was added directly to the biofilm carefully and incubated at 37 °C with 5% CO 2 for 2 h. SNP and DMEM medium were added to control slide biofilms and incubated at 37 °C with 5% CO 2 for 2 h. Slide biofilms were then stained by 0.1 % crystal violet and washed twice with 0.9 % NaCl; the crystal violet-stained biofilms were resuspended in 96 % ethanol, and biofilm cell-associated dye was measured for absorbance at OD 590 nm. To examine whether macrophage-dispersed biofilm cells are phenotypically similar to SNP-dispersed cells, macrophage-, SNP- and DMEM-treated biofilm slides together with the dispersed populations were scraped off the glass slides and loaded into 96-well microplates for the quantification of pyoverdine fluorescence using a microplate reader (Tecan Infinite 2000). C. elegans liquid killing assay To compare the virulence between planktonic and dispersed cells, we used a liquid killing assay with C. elegans as the model host [55] . Planktonic and dispersed bacteria were grown in liquid assay media (2.5 g peptone, 5.0 g tryptone, 2.5 g yeast extract, 5 μg ml −1 cholesterol, 4.0 g NaCl, 7.5 ml glycerol and ddH 2 O in 1 liter) in 96-well microplates. Fifty L4-stage animals were transferred into triplicate wells. The co-cultures were incubated at 25 °C for 6 h and observed for live/dead nematodes under a stereomicroscope (Zeiss). Experiments were performed in triplicate, and the results are shown as the mean±s.d. Iron stress tolerance assay To compare the resistance of planktonic and biofilm-dispersed cells towards iron stress, the growth curves of PAO1 and PAO1/p BAD - yhjH planktonic and dispersed cells were generated in triplicate, as previously described [19] . The cells were adjusted to OD 600 =0.12 and exposed to either ABTGC or ABTGC containing 160 μg ml −1 DIPY. OD 600 measurements were recorded every 15 min for 16 h using a microplate reader (Tecan Infinite 2000) at 37 °C. Experiments were performed in triplicate, and the results are shown as the mean±s.d. Cultivation of PAO1 biofilms in flow chambers Fluorescent-tagged biofilms were cultivated in flow chambers of three channels with dimensions of 40 mm × 4 mm × 1 mm. The flow chamber was assembled as previously described [56] and filled with ABTG medium at 37 °C. The flow channels were each inoculated with 300 μl of 1:1,000 × diluted overnight culture with a syringe and then left without flow for 1 h. Medium flow was started using the Cole-Palmer peristaltic pump with a flow velocity of 0.2 mm s −1 , corresponding to laminar flow with a Reynolds number of 0.02. Three replicate channels were used for each experimental condition. After 72-h growth in the flow channels, PAO1 biofilms were treated with 5 μM SNP; 100 μg ml −1 DIPY; 5 μM SNP and 100 μg ml −1 DIPY; or 5 μM SNP, 100 μg ml −1 DIPY and 10 μg ml −1 tobramycin. PAO1/p BAD - yhjH biofilms were treated with 0.25% arabinose; 100 μg ml −1 DIPY; 0.25% arabinose and 100 μg ml −1 DIPY; or 0.25% arabinose, 100 μg ml −1 DIPY and 10 μg ml −1 tobramycin. After 24 h of treatment, 300 μl aliquots of 20 μM of PI were injected into individual flow channels to stain dead cells in the biofilm. Microscopy and image acquisition of flow chambers All microscopy images were captured and acquired using a Zeiss LSM confocal laser scanning microscope (Carl Zeiss, Germany) with a × 20 objective for monitoring GFP and PI fluorescence. Images were processed using the IMARIS software (Bitplane AG, Switzerland). Quantification of dispersed cells in flow chamber effluent The dispersed cells were collected from the flow chamber effluent after treatment with dispersal agents and DIPY. They were serially diluted, and 100 μl of culture was grown on LB agar plates overnight at 37 °C. The resulting colonies were enumerated, and the CFU ml −1 was calculated. Experiments were performed in triplicate, and the results are shown as the mean±s.d. Accession codes : The RNA-Seq data have been deposited in the NCBI Short Read Archive (SRA) database with accession code SRP041868 . How to cite this article: Chua, S. L. et al. Dispersed cells represent a distinct stage in the transition from bacterial biofilm to planktonic lifestyles. Nat. Commun. 5:4462 doi: 10.1038/ncomms5462 (2014).